BIN1/M-Amphiphysin2 induces clustering of phosphoinositides to recruit its downstream partner dynamin Phosphoinositides play a central role in many physiological processes by assisting the recruitment of proteins to membranes through specific phosphoinositide-binding motifs. How this recruitment is coordinated in space and time is not well understood. Here we show that BIN1/M-Amphiphysin2, a protein involved in T-tubule biogenesis in muscle cells and frequently mutated in centronuclear myopathies, clusters PtdIns(4,5)P 2 to recruit its downstream partner dynamin. By using several mutants associated with centronuclear myopathies, we find that the N-BAR and the SH3 domains of BIN1 control the kinetics and the accumulation of dynamin on membranes, respectively. We show that phosphoinositide clustering is a mechanism shared by other proteins that interact with PtdIns(4,5)P 2 , but do not contain a BAR domain. Our numerical simulations point out that clustering is a diffusion-driven process in which phosphoinositide molecules are not sequestered. We propose that this mechanism plays a key role in the recruitment of downstream phosphoinositide-binding proteins. Amphiphysin1 and 2 (also called BIN1) bind to cellular membranes via a N-terminal BAR domain that dimerizes and forms a positively charged concave surface interacting with the negative charges of the membrane [1] . They also bind via a C-terminal SRC homology 3 (SH3) domain to the proline-rich domain of dynamin. On the basis of these structural features, amphiphysins have been proposed to work as core coordinators during dynamin-mediated vesicle fission [2] , [3] . M-amphiphysin 2 is a splice variant of BIN1 expressed in muscle that has been implicated in T-tubule biogenesis. The exact function of BIN1 is not known but centronuclear myopathies (CNMs), a heterogeneous group of inherited muscular disorders, provide an extreme example in which the function of BIN1 is impaired. Several BIN1 mutations prevent binding to dynamin and result in compromised normal muscle function and nuclei positioning, ultimately leading to fibre atrophy and muscle weakness [4] , [5] . Unlike other amphiphysin isoforms, BIN1 displays a phosphoinositide (PI)-binding domain that is responsible for its targeting to the plasma membrane, mainly by interacting with phosphatidylinositol 4,5-bisphosphate (PtdIns(4,5)P 2 ) [6] . The consequences of BIN1-PtdIns(4,5)P 2 interaction in the selection of downstream partners remain elusive. Here we show using in vitro and in cellulo systems that the N-BAR domain of BIN1 facilitates the recruitment of its downstream partner dynamin by clustering PtdIns(4,5)P 2 , whereas the SH3 domain ensures the accumulation of dynamin at the plasma membrane. We propose that the distinct roles observed for the N-BAR and the SH3 domains of BIN1 may explain why different BIN1 mutations display a similar phenotype in dynamin binding reported in the autosomal form of CNMs. Our work points to PI clustering as a general property of proteins containing N-BAR or PI-interacting motifs (ANTH/ENTH). BIN1 locally recruits PI-binding motifs by clustering PIs To investigate a possible role of BIN1 in the remodelling of PI-containing membranes, we used an in vitro system on the basis of flat membrane sheets with a plasma membrane-like composition containing 2–10% PtdIns(4,5) 2 adapted from [7] ( Fig. 1 ). BAR domain proteins are able to both sense and induce membrane curvature depending on their membrane bound density [8] . For high bulk concentrations (> 1 μM), we observed that BIN1 triggers the formation of dynamic tubules from flat membranes containing 5% PtdIns(4,5)P 2 ( Figs 1 and 2a ). To localize PtdIns(4,5)P 2 after BIN1 membrane binding, we used a PtdIns(4,5)P 2 -binding motif, namely the PH domain from phospholipase Cδ1 (PLCδ1), PH(PLCδ), which displays stereospecific recognition for PtdIns(4,5)P 2 (ref. 9 ) ( Supplementary Fig. 1a ). The binding of PtdIns(4,5)P 2 -binding motif was measured as described in Supplementary Fig. 2 and in the Methods section. We observed that the binding of the motif was increased 47±11-fold in the presence of BIN1 and colocalized to BIN1-positive structures ( Fig. 2b,c and Supplementary Fig. 3a ), compared with control conditions ( Supplementary Fig. 1b,c ). This increase was not observed in the absence of PtdIns(4,5)P 2 , ( Supplementary Fig. 3b ). As expected, a sequential increase in the PtdIns(4,5)P 2 level enhanced the recruitment of the PtdIns(4,5)P 2 -binding motif to membranes ( Fig. 2c , grey boxes). Noteworthy, the amount of PtdIns(4,5)P 2 -binding motif recruited was in any case lower than in the presence of BIN1 on membranes containing 5% PtdIns(4,5)P 2 ( Fig. 1c , green box). 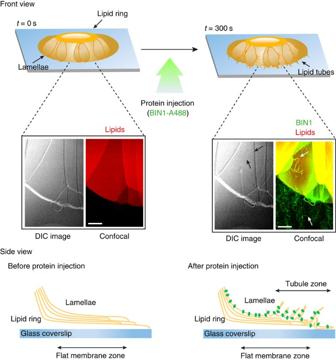Figure 1: Experimental system. The experimentalin vitroset up consists of flat membranes made of a plasma membrane lipid mixture following32, doped with different proportions of PIs and 0.1% red fluorescent GloPIP2. The final lipid mixture is dried, forming a lipid ring. Further addition of buffer leads to the formation of lamellar structures at the boundary of the lipid ring, consisting of several bilayer stacks under low membrane tension. Injection of fluorescently labelled proteins with membrane remodelling activity, such as BIN1 tagged with green AlexaFluor A488, yields the formation of dynamic lipid tubes that emanate from the membranes lamellae (pointed with black and white arrows on the DIC and confocal images, respectively). After BIN1 addition, two distinct zones can be distinguished: the ‘flat membrane zone’ closer to the lipid ring and the ‘tubule zone’ at the rim of the lamellae from which BIN1-induced tubules form (see the side view drawings where BIN1 is represented by green ovals). Note that independently of the proportion of PIs used, (i) the flat membranes contain 0.1% of fluorescent PtdIns(4,5)P2(Glo-PIP2) and (ii) BIN1 can only bind to the outermost lipid bilayer. Because lamella regions on flat membranes contain several bilayer stacks, the membrane fluorescence intensity in the flat membrane zone is higher than in the tubule zone in which lipid tubes obtained after BIN1 addition are formed by a single bilayer. As a result, all fluorescence intensity measurements (see Methods) were normalized by the membrane intensity of the region of interest, to correct for the heterogeneous distribution of membrane stacks throughout the sample. Scale bars, 20 μm. Figure 1: Experimental system. The experimental in vitro set up consists of flat membranes made of a plasma membrane lipid mixture following [32] , doped with different proportions of PIs and 0.1% red fluorescent GloPIP 2 . The final lipid mixture is dried, forming a lipid ring. Further addition of buffer leads to the formation of lamellar structures at the boundary of the lipid ring, consisting of several bilayer stacks under low membrane tension. Injection of fluorescently labelled proteins with membrane remodelling activity, such as BIN1 tagged with green AlexaFluor A488, yields the formation of dynamic lipid tubes that emanate from the membranes lamellae (pointed with black and white arrows on the DIC and confocal images, respectively). After BIN1 addition, two distinct zones can be distinguished: the ‘flat membrane zone’ closer to the lipid ring and the ‘tubule zone’ at the rim of the lamellae from which BIN1-induced tubules form (see the side view drawings where BIN1 is represented by green ovals). Note that independently of the proportion of PIs used, (i) the flat membranes contain 0.1% of fluorescent PtdIns(4,5)P 2 (Glo-PIP 2 ) and (ii) BIN1 can only bind to the outermost lipid bilayer. Because lamella regions on flat membranes contain several bilayer stacks, the membrane fluorescence intensity in the flat membrane zone is higher than in the tubule zone in which lipid tubes obtained after BIN1 addition are formed by a single bilayer. As a result, all fluorescence intensity measurements (see Methods) were normalized by the membrane intensity of the region of interest, to correct for the heterogeneous distribution of membrane stacks throughout the sample. Scale bars, 20 μm. 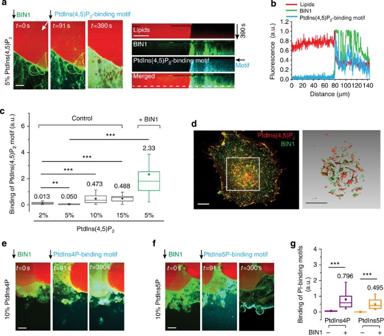Figure 2: BIN1 locally recruits PI-binding motifs. (a) Recruitment of 1 μM of PtdIns(4,5)P2-binding motif (PH(PLCδ)) to 5% PtdIns(4,5)P2membranes after incubation with 2 μM BIN1. Kymograph obtained along the diagonal from the top right corner (white arrow). (b) Intensity profile along the white dashed lines in the kymographa. (c) Binding of the PtdIns(4,5)P2-binding motif to flat membranes under increasing amounts of PtdIns(4,5)P2without BIN1 (grey) and in the presence of 2 μM BIN1 at 5% PtdIns(4,5)P2(green). (d) HeLa cells co-expressing GFP-BIN1 and mCherry-PH(PLCδ) (see Methods). (e,f) Still images showing the recruitment of 1 μM PI-binding motifs to PI-containing membranes after incubation with 2 μM BIN1 (e, PH(OSH2) to 10% PtdIns4P membranes,f, PHD(ING2) to 10% PtdIns5P membranes). (g) Binding of the PI-binding motifs to flat membranes in the presence or absence of 2 μM BIN1 (±BIN1) for PtdIns4P and PtdIns5P. Scale bars, 20 μm forin vitroassays, 10 μm for cell imaging. Measurements were performed from at least three independent experiments. Box plots display the average value (solid square, also shown on top of each box plot), the median value (solid line), the s.d. and the interquartile range (25–75%) (n=23,n=39,n=30,n=23 andn=35, for control at 2%, 5%, 10%, 15% PtdIns(4,5)P2, and+BIN1 at 5% PtdIns(4,5)P2, respectively.n=22,n=25,n=24 andn=24 for PtdIns4P in control and+BIN1, and PtdIns5P in control and+BIN1, respectively). Error bars represent s.d. **P<0.01, ***P<0.001 (t-test). Full size image Figure 2: BIN1 locally recruits PI-binding motifs. ( a ) Recruitment of 1 μM of PtdIns(4,5)P 2 -binding motif (PH(PLCδ)) to 5% PtdIns(4,5)P 2 membranes after incubation with 2 μM BIN1. Kymograph obtained along the diagonal from the top right corner (white arrow). ( b ) Intensity profile along the white dashed lines in the kymograph a . ( c ) Binding of the PtdIns(4,5)P 2 -binding motif to flat membranes under increasing amounts of PtdIns(4,5)P 2 without BIN1 (grey) and in the presence of 2 μM BIN1 at 5% PtdIns(4,5)P 2 (green). ( d ) HeLa cells co-expressing GFP-BIN1 and mCherry-PH(PLCδ) (see Methods). ( e , f ) Still images showing the recruitment of 1 μM PI-binding motifs to PI-containing membranes after incubation with 2 μM BIN1 ( e , PH(OSH2) to 10% PtdIns4P membranes, f , PHD(ING2) to 10% PtdIns5P membranes). ( g ) Binding of the PI-binding motifs to flat membranes in the presence or absence of 2 μM BIN1 (±BIN1) for PtdIns4P and PtdIns5P. Scale bars, 20 μm for in vitro assays, 10 μm for cell imaging. Measurements were performed from at least three independent experiments. Box plots display the average value (solid square, also shown on top of each box plot), the median value (solid line), the s.d. and the interquartile range (25–75%) ( n =23, n =39, n =30, n =23 and n =35, for control at 2%, 5%, 10%, 15% PtdIns(4,5)P 2 , and+BIN1 at 5% PtdIns(4,5)P 2 , respectively. n =22, n =25, n =24 and n =24 for PtdIns4P in control and+BIN1, and PtdIns5P in control and+BIN1, respectively). Error bars represent s.d. ** P <0.01, *** P <0.001 ( t -test). Full size image From the data in Fig. 2c , we estimated that the PI enrichment assisted by BIN1 represents at least a threefold increase in the local PtdIns(4,5)P 2 concentration (that is, over 15% of the total amount of total lipids, under our experimental conditions). To confirm that it was also the case in cellulo , we overexpressed BIN1 in HeLa cells. As previously reported, overexpression of BIN1 induces the formation of tubules, mostly emanating from the plasma membrane towards the inside of the cells [4] , [6] , [10] . In agreement to what we observed in vitro , our in cellulo data showed a high accumulation of PtdIns(4,5)P 2 in BIN1-positive structures as compared with control conditions ( Fig. 2d and Supplementary Fig. 4 ). The PI-binding domain of BIN1 also interacts with other PIs, including PtdIns4P and PtdIns5P (refs 5 , 6 ), although to a lower affinity than to PtdIns(4,5)P 2 ( Supplementary Fig. 5 ). We observed that BIN1 (> 1 μM) induces membrane deformation in flat membranes containing at least 10% of PtdIns4P or PtdIns5P. The recruitment of PtdIns4P- and PtdIns5P-binding motifs, namely the PH domain of OSH2 (ref. 11 ) (PH(OSH2)) and the PHD-finger of ING2 (ref. 12 ) (PHD(ING2)), respectively, was enhanced in the presence of BIN1 and accumulated in BIN1-positive structures ( Fig. 2e–g , Supplementary Fig. 1a,d–g , and Supplementary Fig. 3c,d , red arrows). Altogether, these results suggest that BIN1 has the capability to accumulate PIs and thus, to locally recruit different PI-binding motifs to membranes. In the following, we refer to the accumulation of PIs as PI clustering. Dynamin recruitment depends on PI clustering induced by BIN1 We then investigated the role of PI-clustering induced by BIN1 in the recruitment of downstream partners. To this aim, we focused on dynamin recruitment using our in vitro system ( Fig. 1 ). Previous studies have shown that curvature has a pivotal role in dynamin function as its polymerization only occurs above a threshold in membrane curvature [13] . To distinguish the effects of BIN1-induced PtdIns(4,5)P 2 clustering from that of curvature sensing in dynamin recruitment, we worked with 0.3 μM dynamin, a concentration at which experimental data reported that dynamin does not polymerize [13] . Binding of dynamin to flat membranes clearly depended on the amount of PtdIns(4,5)P 2 ( Fig. 3a,b and Supplementary Fig. 6a–c ). As a result, no dynamin binding was observed below 2% PtdIns(4,5)P 2 and only weak binding at 5% PtdIns(4,5)P 2 . A 10-fold increase in dynamin binding occurred at 10% PtdIns(4,5)P 2 , probably reflecting dynamin polymerization ( Fig. 3b ). Moreover, the kinetics of dynamin recruitment followed a cooperative behaviour, consistent with the dimeric (K D >1 mM) and oligomeric (K D >9 μM) states of dynamin [14] ( Supplementary Fig. 6d ). Remarkably, in the presence of BIN1, dynamin binding to membranes containing 5% PtdIns(4,5)P 2 was increased 42±13-fold with a 2.4-fold faster kinetics ( Fig. 3b,c,e ). 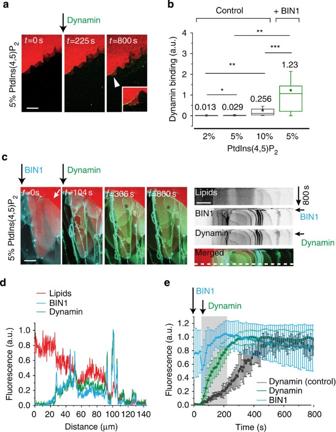Figure 3: Dynamin recruitment to PI-containing membranes is enhanced by BIN1. (a) Binding of 0.3 μM dynamin to 5% PtdIns(4,5)P2flat membranes. A region showing local dynamin binding is highlighted with a white arrow and in image inset. (b) Binding of 0.3 μM dynamin to flat membranes containing 2%, 5% and 10% PtdIns(4,5)P2, respectively, and at 5% PtdIns(4,5)P2in the presence of 2 μM BIN1. (c) Binding of 0.3 μM dynamin to flat membranes containing 5% PtdIns(4,5)P2previously incubated with 2 μM BIN1. Kymograph obtained along the diagonal from the top right corner. (d) Intensity profile along the white dashed line in the kymograph. (e) Binding kinetics of 0.3 μM dynamin to flat membranes containing 5% PtdIns(4,5)P2in control conditions and in the presence of 2 μM BIN1 (cyan curve). The shadowed region highlights the rise in BIN1 fluorescence after dynamin addition. Measurements were performed from at least three independent experiments. Box plots display the average value (solid square, also shown on top of each box plot), the median value (solid line), the s.d. and the interquartile range (25–75%) (n=14,n=15,n=21 andn=37, for control at 2%, 5%, 10%, PtdIns(4,5)P2and+BIN1 at 5% PtdIns(4,5)P2, respectively). Error bars represent s.d. *P<0.1, **P<0.01, ***P<0.001 (t-test). Scale bars, 20 μm. Figure 3: Dynamin recruitment to PI-containing membranes is enhanced by BIN1. ( a ) Binding of 0.3 μM dynamin to 5% PtdIns(4,5)P 2 flat membranes. A region showing local dynamin binding is highlighted with a white arrow and in image inset. ( b ) Binding of 0.3 μM dynamin to flat membranes containing 2%, 5% and 10% PtdIns(4,5)P 2 , respectively, and at 5% PtdIns(4,5)P 2 in the presence of 2 μM BIN1. ( c ) Binding of 0.3 μM dynamin to flat membranes containing 5% PtdIns(4,5)P 2 previously incubated with 2 μM BIN1. Kymograph obtained along the diagonal from the top right corner. ( d ) Intensity profile along the white dashed line in the kymograph. ( e ) Binding kinetics of 0.3 μM dynamin to flat membranes containing 5% PtdIns(4,5)P 2 in control conditions and in the presence of 2 μM BIN1 (cyan curve). The shadowed region highlights the rise in BIN1 fluorescence after dynamin addition. Measurements were performed from at least three independent experiments. Box plots display the average value (solid square, also shown on top of each box plot), the median value (solid line), the s.d. and the interquartile range (25–75%) ( n =14, n =15, n =21 and n =37, for control at 2%, 5%, 10%, PtdIns(4,5)P 2 and+BIN1 at 5% PtdIns(4,5)P 2 , respectively). Error bars represent s.d. * P <0.1, ** P <0.01, *** P <0.001 ( t -test). Scale bars, 20 μm. Full size image Colocalization of dynamin to BIN1-positive structures confirmed that BIN1 is implicated in the spatiotemporal recruitment of dynamin to membranes (see the corresponding fluorescence signal in the kymograph cross-section, Fig. 3d ) and that membrane remodelling induced by BIN1 might have a decisive upstream role in dynamin recruitment. In addition, we observed a rise in BIN1 fluorescent signal on dynamin binding (grey shadow in Fig. 3e ). This observation suggests a positive feedback recruitment of the two proteins, a behaviour already reported for N-BAR proteins at high PtdIns(4,5)P 2 concentrations [15] . To further determine whether dynamin is recruited owing to the high local concentration of PtdIns(4,5)P 2 generated by BIN1 or to its curvature sensing ability, we monitored dynamin binding in samples in which BIN1 did not induce lipid-tube formation. This happens when membranes do not detach from the lipid reservoir, and thus remain under tension. As shown in Fig. 4a,b , a 9±4-fold in dynamin binding was still observed in the absence of BIN1-induced membrane tubulation, suggesting that dynamin recruitment is not only due to its curvature sensing ability, but also due to PtdIns(4,5)P 2 clustering by BIN1. To further confirm this hypothesis, we performed experiments at very low concentration of dynamin (0.1 μM, well below the concentration required for dynamin polymerization on BIN1-induced tubules) on membranes containing 5% PtdIns(4,5)P 2 . Under these conditions, a 6±2-fold increase in dynamin binding was observed in the presence of BIN1 ( Fig. 4c ). Altogether, the above results suggest that, once a critical value in dynamin polymerization is reached, the accumulation of dynamin on BIN1-positive tubules as a result of PI clustering is further increased either due to the curvature sensing properties of dynamin or due to a positive feedback mechanism (or a combination of both). 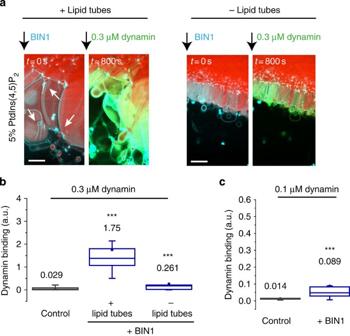Figure 4: Dynamin recruitment on membranes depends on BIN1-induced PtdIns(4,5)P2clustering. (a,b) Binding of 0.3 μM dynamin (green) to flat membranes containing 5% PtdIns(4,5)P2either displaying lipid tubes (white arrows, left panel) or not (right panel) after BIN1 injection (cyan). (c) Binding of 0.1 μM dynamin to flat membranes containing 5% PtdIns(4,5)P2after BIN1 injection. Measurements were performed from at least three independent experiments (n=15,n=24 andn=13, for 0.3 μM dynamin in control conditons, +lipid tubes, and −lipid tubes, respectively.n=13 andn=21 for 0.1 μM dynamin in control conditons and+BIN1, respectively). Box plots display the average value (solid square, also shown on top of each box plot), the median value (solid line), the s.d. and the interquartile range (25–75%). Error bars represent s.d. ***P<0.001 (t-test). Error bars represent s.d.. Scale bars, 20 μm. Figure 4: Dynamin recruitment on membranes depends on BIN1-induced PtdIns(4,5)P 2 clustering. ( a , b ) Binding of 0.3 μM dynamin (green) to flat membranes containing 5% PtdIns(4,5)P 2 either displaying lipid tubes (white arrows, left panel) or not (right panel) after BIN1 injection (cyan). ( c ) Binding of 0.1 μM dynamin to flat membranes containing 5% PtdIns(4,5)P 2 after BIN1 injection. Measurements were performed from at least three independent experiments ( n =15, n =24 and n =13, for 0.3 μM dynamin in control conditons, +lipid tubes, and −lipid tubes, respectively. n =13 and n =21 for 0.1 μM dynamin in control conditons and+BIN1, respectively). Box plots display the average value (solid square, also shown on top of each box plot), the median value (solid line), the s.d. and the interquartile range (25–75%). Error bars represent s.d. *** P <0.001 ( t -test). Error bars represent s.d.. Scale bars, 20 μm. Full size image The N-BAR and the SH3 domains of BIN1 display distinct roles We next evaluated the relative contribution of PtdIns(4,5)P 2 clustering and that of the interaction between the SH3 domain of BIN1 and the proline-rich domain of dynamin [16] in the recruitment of dynamin on membranes. To this aim, we compared the ability of full-length BIN1, amphiphysin1 (that does not contain a PI-binding domain) and of BIN1 SH3-ΔC (a mutated variant of BIN1 found in an autosomal recessive form of CNMs that displays a truncated SH3 domain [17] ) ( Fig. 5a ) to recruit dynamin. The three proteins speeded up the rate of dynamin recruitment by a factor 2.35±0.05, 1.59±0.04 and 2.27±0.04, respectively as compared with control conditions ( Fig. 5b ). BIN1 and amphiphysin1 increased the binding of dynamin to membranes by 43±13- and 54±16-fold, respectively ( Fig. 5c ). Importantly, an increase in dynamin binding could also be detected in the presence of BIN1 SH3-ΔC, although to a lower extent (14±4-fold). To further support the contribution of PtdIns(4,5)P 2 clustering to dynamin binding, we compared the impact on dynamin recruitment of a BIN1 construct containing only the N-BAR domain to that of a construct carrying a mutation in the N-BAR domain (N-BAR D151N) found in CNMs [4] and that does not deform membranes [18] ( Fig. 5a ). As expected, the lack of the SH3 domain led to a lower dynamin accumulation on membranes for both constructs ( Fig. 5c ). However, in the presence of the N-BAR domain, dynamin exhibited a similar binding kinetics to that observed in the presence of full-length BIN1 or amphiphysin1 ( Fig. 5b , lower and middle panel, respectively). In contrast, the N-BAR D151N displayed kinetics of dynamin recruitment comparable to that observed with dynamin alone ( Fig. 5b , lower panel). In addition, the BIN1 N-BAR domain was able to cluster PtdIns(4,5)P 2 to a much larger extent than the N-BAR D151N mutant ( Fig. 6a,b ). This suggests that PtdIns(4,5)P 2 clustering induced by the N-BAR domain controls the kinetics of dynamin recruitment independently of the SH3 domain. 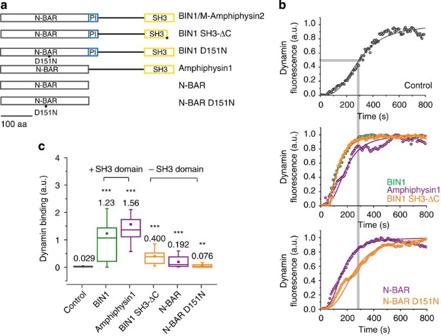Figure 5: The N-BAR and SH3 domains of BIN1 have distinct roles in the recruitment of dynamin. (a) Domain representation (N-BAR, PI domain and SH3 domain) of the full-length and N-BAR domain constructs used. Mutated amino acids in N-BAR D151N and stop codon in BIN1 SH3-ΔC are highlighted with a black star. (b) Binding kinetics of 0.3 μM dynamin to flat membranes containing 5% PtdIns(4,5)P2in control conditions (dynamin alone) and in the presence of the constructs described in panela. Data were fitted (solid lines) as described in Methods. (c) Binding of 0.3 μM dynamin to flat membranes containing 5% PtdIns(4,5)P2in control conditions and in the presence of the constructs described in panela. Measurements were performed from at least three independent experiments. Box plots display the average value (solid square, also shown on top of each box plot), the median value (solid line), the s.d. and the interquartile range (25–75%) (n=15,n=37,n=29,n=24,n=22 andn=31, for control, BIN1, Amphiphysin1, BIN1 SH3-ΔC, N-BAR, N-BAR D151N, respectively). Error bars represent s.d. **P<0.01, ***P<0.001 (t-test). Figure 5: The N-BAR and SH3 domains of BIN1 have distinct roles in the recruitment of dynamin. ( a ) Domain representation (N-BAR, PI domain and SH3 domain) of the full-length and N-BAR domain constructs used. Mutated amino acids in N-BAR D151N and stop codon in BIN1 SH3-ΔC are highlighted with a black star. ( b ) Binding kinetics of 0.3 μM dynamin to flat membranes containing 5% PtdIns(4,5)P 2 in control conditions (dynamin alone) and in the presence of the constructs described in panel a . Data were fitted (solid lines) as described in Methods. ( c ) Binding of 0.3 μM dynamin to flat membranes containing 5% PtdIns(4,5)P 2 in control conditions and in the presence of the constructs described in panel a . Measurements were performed from at least three independent experiments. Box plots display the average value (solid square, also shown on top of each box plot), the median value (solid line), the s.d. and the interquartile range (25–75%) ( n =15, n =37, n =29, n =24, n =22 and n =31, for control, BIN1, Amphiphysin1, BIN1 SH3-ΔC, N-BAR, N-BAR D151N, respectively). Error bars represent s.d. ** P <0.01, *** P <0.001 ( t -test). 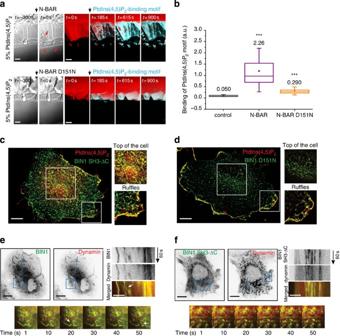Figure 6: The N-BAR domain is responsible for PI clustering. (a) Binding of the PtdIns(4,5)P2-binding motif PH(PLCδ) (in cyan) on flat membranes containing 5% PtdIns(4,5)P2(0.1% GloPIP2, in red) previously incubated with 2 μM of the BIN1 N-BAR or 2 μM of the BIN1-mutated N-BAR D151N. Red arrows point to the formation of membrane tubes after N-BAR incubation. (b) Binding of the PtdIns(4,5)P2motif PH(PLCδ) to flat membranes containing 5% PtdIns(4,5)P2in control conditions (grey) and in the presence of the N-BAR domain (magenta) or the N-BAR D151N (orange). (c,d) HeLa cells co-expressing GFP-BIN1 SH3-ΔC (c) or GFP-BIN1 D151N (d) mutants along with mCherry-PH(PLCδ) (see Methods). (e,f) Live-cell imaging (500 ms for 60 s) of HeLa cells co-expressing GFP-BIN1 (e) or GFP-BIN1 SH3-ΔC (f) together with mCherry-dynamin (see Methods). White arrows point to fission events observed in (e). Kymographs were obtained along the blue lines. Measurements were performed from at least three independent experiments. Box plots display the average value (solid square, also shown on top of each box plot), the median value (solid line), the s.d. and the interquartile range (25–75%) (n=39,n=27 andn=22, for control, N-BAR and N-BAR D151N, respectively). Error bars represent s.d. ***P<0.001 (t-test). Scale bars, 20 μm for flat membranes, 10 μm for cell imaging and 2 μm for kymographs. Full size image Figure 6: The N-BAR domain is responsible for PI clustering. ( a ) Binding of the PtdIns(4,5)P 2 -binding motif PH(PLCδ) (in cyan) on flat membranes containing 5% PtdIns(4,5)P 2 (0.1% GloPIP2, in red) previously incubated with 2 μM of the BIN1 N-BAR or 2 μM of the BIN1-mutated N-BAR D151N. Red arrows point to the formation of membrane tubes after N-BAR incubation. ( b ) Binding of the PtdIns(4,5)P 2 motif PH(PLCδ) to flat membranes containing 5% PtdIns(4,5)P 2 in control conditions (grey) and in the presence of the N-BAR domain (magenta) or the N-BAR D151N (orange). ( c , d ) HeLa cells co-expressing GFP-BIN1 SH3-ΔC ( c ) or GFP-BIN1 D151N ( d ) mutants along with mCherry-PH(PLCδ) (see Methods). ( e , f ) Live-cell imaging (500 ms for 60 s) of HeLa cells co-expressing GFP-BIN1 ( e ) or GFP-BIN1 SH3-ΔC ( f ) together with mCherry-dynamin (see Methods). White arrows point to fission events observed in ( e ). Kymographs were obtained along the blue lines. Measurements were performed from at least three independent experiments. Box plots display the average value (solid square, also shown on top of each box plot), the median value (solid line), the s.d. and the interquartile range (25–75%) ( n =39, n =27 and n =22, for control, N-BAR and N-BAR D151N, respectively). Error bars represent s.d. *** P <0.001 ( t -test). Scale bars, 20 μm for flat membranes, 10 μm for cell imaging and 2 μm for kymographs. Full size image To confirm the above results in cellulo , we expressed in HeLa cells full-length BIN1, D151N and SH3-ΔC mutants ( Fig. 5a ). We observed that whereas the SH3-ΔC mutant accumulates PtdIns(4,5)P 2 in BIN1-positive structures ( Fig. 6c ), the D151N mutant did not ( Fig. 6d ), in agreement with our in vitro data. We then investigated the ability of the BIN1 SH3-ΔC mutant to recruit dynamin. Live imaging experiments in cells co-expressing either BIN1 or the BIN1 SH3-ΔC mutant along with dynamin revealed that both proteins are capable to recruit dynamin to BIN1-positive structures ( Fig. 6e,f ), likely through PtdIns(4,5)P 2 clustering (previously shown in Figs 2d and 6c , respectively). Interestingly, fission events were only observed in BIN1/dynamin-positive structures (white arrows in Fig. 6e , and Supplementary Movie 1 ) but not in BIN1 SH3-ΔC/dynamin-positive structures ( Fig. 6f and Supplementary Movie 2 ). Together, these results demonstrate a separate role for the N-BAR domain, which controls the kinetics, and the SH3 domain of BIN1, which ensures dynamin accumulation on membranes. PI clustering is also a property of ANTH and ENTH domains To investigate whether PtdIns(4,5)P 2 clustering could be a general mechanism and to evaluate the contribution of membrane curvature to this process, we next monitored the binding of two other proteins that interact with PtdIns(4,5)P 2 , namely AP180 and Epsin2 (ref. 19 ). Notably, whereas the ENTH domain of Epsin2 triggers membrane deformation by inserting its N-terminal helix into the membrane [20] , the ANTH domain of AP180 does not induce curvature [21] . Using our in vitro system ( Fig. 1 ), we observed an increased accumulation of PtdIns(4,5)P 2 -binding motifs in both Epsin2 and AP180-positive structures on membranes containing 5% PtdIns(4,5)P 2 ( Fig. 7a,b , see red arrows and Supplementary Fig. 7a,b ). This effect was more pronounced for Epsin2 (ENTH domain) than for AP180 (ANTH domain) ( Fig. 7c–e ), with a 33±8-fold and 20±4-fold increase, respectively. This suggests that PtdIns(4,5)P 2 clustering might be a general property of proteins that, like BIN1, interact with PIs (that is, Epsin2 and AP180) and that curvature amplifies this effect. Using liposome flotation assays, we observed that the binding of the PH(PLCδ) used as PtdIns(4,5)P 2 -binding motif was sensitive to membrane curvature, although to a much lesser extent than curvature sensors such as ALPS motifs [22] . This curvature sensitivity was dependent on the concentration of the probe, being more pronounced on ~30-nm liposomes at low PH(PLCδ) concentrations ( Supplementary Fig. 8 ) This suggests that rather than curvature sensing, the lipid defects associated with membrane curvature might enhance the interaction between PtdIns(4,5)P 2 headgroups and the PtdIns(4,5)P 2 -binding motif of PH(PLCδ). 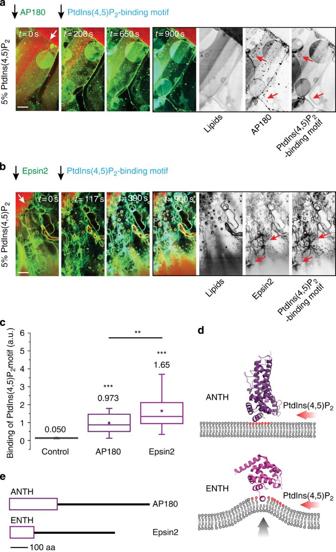Figure 7: ANTH and ENTH domains recruit PtdIns(4,5)P2-binding motif. (a,b) Recruitment of the PtdIns(4,5)P2-binding motif (PH(PLCδ)) to 5% PtdIns(4,5)P2flat membranes previously incubated with 2 μM AP180 (a) or 2 μM Epsin2 (b). (c) Binding of the PtdIns(4,5)P2-motif to 5% PtdIns(4,5)P2flat membranes in control conditions and in the presence of 2 μM AP180 or 2 μM Epsin2. (d) Formation of PtdIns(4,5)P2clusters through the interaction of the ANTH and ENTH domains with PtdIns(4,5)P2-containing membranes. (e) Domain representation of the ANTH domain of AP180 and the ENTH domain of Epsin2. Measurements were performed from at least three independent experiments. Box plots display the average value (solid square, also shown on top of each box plot), the median value (solid line) the s.d. and the interquartile range (25–75%) (n=39,n=35 andn=31, for control, AP180 and Epsin2, respectively). Error bars represent s.d. ***P<0.001 (t-test). Scale bars, 20 μm. Figure 7: ANTH and ENTH domains recruit PtdIns(4,5)P 2 -binding motif. ( a , b ) Recruitment of the PtdIns(4,5)P 2 -binding motif (PH(PLCδ)) to 5% PtdIns(4,5)P 2 flat membranes previously incubated with 2 μM AP180 ( a ) or 2 μM Epsin2 ( b ). ( c ) Binding of the PtdIns(4,5)P 2 -motif to 5% PtdIns(4,5)P 2 flat membranes in control conditions and in the presence of 2 μM AP180 or 2 μM Epsin2. ( d ) Formation of PtdIns(4,5)P 2 clusters through the interaction of the ANTH and ENTH domains with PtdIns(4,5)P 2 -containing membranes. ( e ) Domain representation of the ANTH domain of AP180 and the ENTH domain of Epsin2. Measurements were performed from at least three independent experiments. Box plots display the average value (solid square, also shown on top of each box plot), the median value (solid line) the s.d. and the interquartile range (25–75%) ( n =39, n =35 and n =31, for control, AP180 and Epsin2, respectively). Error bars represent s.d. *** P <0.001 ( t -test). Scale bars, 20 μm. Full size image Modelling of PI clustering on membranes We estimated that the binding of the N-BAR domain or the ANTH/ENTH domain on PI-containing membranes results in a local increase of at least three times the initial amount of PtdIns(4,5)P 2 (compare the binding of the PI-binding motif on membranes containing 15% PtdIns(4,5)P 2 in the absence of proteins with the binding of the PI-binding motif on membranes containing 5% PtdIns(4,5)P 2 in the presence of BIN1, AP180 and Epsin2 from Figs 2c and 7c ). How such PtdIns(4,5)P 2 enrichment can be reached? The charge and area of a N-BAR homodimer are +8e and 50 nm 2 and that of a PtdIns(4,5)P 2 molecule are −4e and 0.68 nm 2 , respectively [1] , [23] . A simple stoichiometric argument on the basis of the number of PtdIns(4,5)P 2 molecules [23] with which a N-BAR homodimer interacts [1] (that is, two) leads to a 1.5-fold enrichment, a value that is below the local PtdIns(4,5)P 2 enrichment observed in our experiments. To see whether this enrichment could be explained by local PtdIns(4,5)P 2 demixing, we resorted to quasi-atomistic coarse grain (CG) molecular dynamics (MD) simulations to investigate the molecular mechanism of membrane binding of the N-BAR and ANTH/ENTH domains. In our in silico systems, a single copy of each protein domain was initially positioned between 6 and 10 nm away from a lipid bilayer containing PtdIns(4,5)P 2 lipids at a 5% mol concentration. Multiple independent simulations were performed to study its spontaneous partitioning and the subsequent reorganization of PtdIns(4,5)P 2 molecules. In all cases, the protein bound to the bilayer and induced PtdIns(4,5)P 2 clustering, as shown by both PtdIns(4,5)P 2 density in the protein proximity ( Fig. 8a ) and by the radial distribution function of PtdIns(4,5)P 2 molecules around the protein ( Supplementary Fig. 9 ). As a control, no clustering was observed neither for PtdIns(4,5)P 2 molecules in the opposite leaflet nor for other membrane lipids ( Supplementary Fig. 9 ). 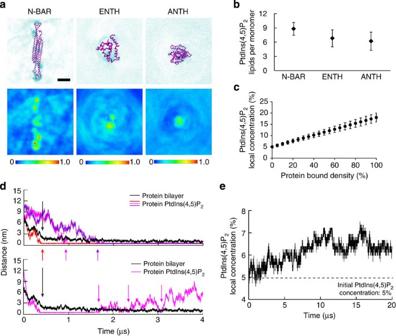Figure 8: PtdIns(4,5)P2remodelling on protein binding is a diffusion-driven process. (a) Top view of PtdIns(4,5)P2clustering in MD simulations on spontaneous membrane binding of N-BAR (left), ENTH (middle) and ANTH (right) domains. In the top panels, a single snapshot of the three proteins are shown in magenta, whereas the individual position of all PtdIns(4,5)P2lipids along the trajectory are shown in cyan. Bottom panels: cumulative PtdIns(4,5)P2area density along the trajectory. (b) Average number of bound PtdIns(4,5)P2molecules per monomer as computed from the final snapshots of five independent 4 μs long MD simulations for each protein. (c) Expected PtdIns(4,5)P2local concentration as a function of membrane-bound protein density in the case of the N-BAR homodimer (see Methods). (d) Representative time traces of the ENTH-membrane distance along the membrane normal (black) and of the minimum distance between ENTH and individual PtdIns(4,5)P2lipids in the membrane plane (colours). Protein binding takes place after ~500 ns, and (i) lipid-binding events can occur simultaneously (red) or after (magenta, violet) membrane binding (top panel) and (ii) dissociation events between the protein and bound PtdIns(4,5)P2lipids can also be observed (bottom panel). An analogous behaviour is observed for ANTH and N-BAR proteins. (e) Time evolution of PtdIns(4,5)P2local concentration in the half of the simulation box in which the diffusion of the N-BAR homodimer was confined. Initial concentration: 5% PtdIns(4,5)P2. Scale bar, 4 nm. Error bars represent s.d. Figure 8: PtdIns(4,5)P 2 remodelling on protein binding is a diffusion-driven process. ( a ) Top view of PtdIns(4,5)P 2 clustering in MD simulations on spontaneous membrane binding of N-BAR (left), ENTH (middle) and ANTH (right) domains. In the top panels, a single snapshot of the three proteins are shown in magenta, whereas the individual position of all PtdIns(4,5)P 2 lipids along the trajectory are shown in cyan. Bottom panels: cumulative PtdIns(4,5)P 2 area density along the trajectory. ( b ) Average number of bound PtdIns(4,5)P 2 molecules per monomer as computed from the final snapshots of five independent 4 μs long MD simulations for each protein. ( c ) Expected PtdIns(4,5)P 2 local concentration as a function of membrane-bound protein density in the case of the N-BAR homodimer (see Methods). ( d ) Representative time traces of the ENTH-membrane distance along the membrane normal (black) and of the minimum distance between ENTH and individual PtdIns(4,5)P 2 lipids in the membrane plane (colours). Protein binding takes place after ~500 ns, and (i) lipid-binding events can occur simultaneously (red) or after (magenta, violet) membrane binding (top panel) and (ii) dissociation events between the protein and bound PtdIns(4,5)P 2 lipids can also be observed (bottom panel). An analogous behaviour is observed for ANTH and N-BAR proteins. ( e ) Time evolution of PtdIns(4,5)P 2 local concentration in the half of the simulation box in which the diffusion of the N-BAR homodimer was confined. Initial concentration: 5% PtdIns(4,5)P 2 . Scale bar, 4 nm. Error bars represent s.d. Full size image In the simulations, all protein domains induced PtdIns(4,5)P 2 clustering ( Fig. 8b ), with up to nine PtdIns(4,5)P 2 lipids bound per monomer in the case of the N-BAR domain. As a result, on protein binding, the local PtdIns(4,5)P 2 concentration can reach 15–20%, depending on the membrane density of the bound protein ( Fig. 8c ), consistent with our in vitro observations of a threefold increase in local PtdIns(4,5)P 2 concentration ( Fig. 2c ). As the observed number of PtdIns(4,5)P 2 lipids per protein ( Fig. 8b ) is larger than the number of PtdIns(4,5)P 2 protein-binding sites, the clustering of PtdIns(4,5)P 2 appears to be primarily driven by non-specific electrostatic interactions. To test this hypothesis, we replaced the BAR, ENTH or ANTH domains with short polylysine motifs (unstructured loops composed of eight lysine residues) in our simulations. In the presence of polylysine motifs, we also observed PtdIns(4,5)P 2 clustering, thus confirming the crucial role of non-specific electrostatic interactions ( Supplementary Fig. 10 ). This observation also justifies a posteriori the chosen CG methodology; even though the MARTINI force field has been shown to be able to accurately model the spontaneous recognition of PIs by peripheral proteins [24] , CG models have intrinsic limitations with regard to the study of specific protein–lipid interactions. In this case, however, the model reproduces well the experimental observations because of the non-specific electrostatic interactions underlying the binding mechanism. Next, we focused on the PtdIns(4,5)P 2 -clustering mechanism. Even though membrane partitioning and PtdIns(4,5)P 2 binding may occur simultaneously, most of the PtdIns(4,5)P 2 segregation took place after the protein was already bound to the bilayer ( Fig. 8d and Supplementary Fig. 11 ). Remarkably, we also observed several protein-PtdIns(4,5)P 2 dissociation events ( Fig. 8d and Supplementary Fig. 11 ), indicating that PtdIns(4,5)P 2 molecules are not sequestered and thus available for the recruitment of secondary downstream proteins, such as dynamin. To further confirm the role of lipid diffusion in PtdIns(4,5)P 2 clustering, we designed a new in silico assay in which we doubled the area of the membrane patch in the MD simulations, and we confined protein diffusion in one half of the simulation box (see Methods). By monitoring the number of PtdIns(4,5)P 2 molecules in the half of the membrane patch in which the protein was confined, we observed an increase in PtdIns(4,5)P 2 concentration ( Fig. 8e ) that is consistent with the predicted concentration as a function of membrane density ( Fig. 8c ), considering that the protein-bound density is of ~10% in our MD simulations. The same behaviour was also observed at a lower initial PtdIns(4,5)P 2 concentration ( Supplementary Fig. 12 ). Our work shows that BIN1 can cluster PIs in vitro , including PtdIns4P, PtdIns5P and PtdIns(4,5)P 2 ( Fig. 2 ). The accumulation of PtdIns(4,5)P 2 in BIN1-positive structures in cellulo ( Fig. 2d ) suggests that BIN1 also clusters PIs in cells. We wondered whether this local increase in PI concentration could be involved in the selection of downstream partners of BIN1. Our data show that PI clustering induced by the N-BAR domain of BIN1 controls the kinetics of dynamin recruitment, whereas its SH3 domain is decisive to further ensure dynamin accumulation on membranes, likely facilitating subsequent dynamin polymerization ( Fig. 5 ). The fact that a nine fold increase in dynamin binding was observed in samples where BIN1 does not induce membrane curvature, compared with a ≥40-fold increase on curved membranes ( Fig. 4 ), reveals the complex interplay between PtdIns(4,5)P 2 clustering and membrane curvature. In addition to the SH3-proline-rich domain interaction, membrane curvature likely regulates the optimal conditions for dynamin polymerization on membranes ( Figs 4 and 5 ). Extrapolating our results on BIN1 to endophilin, this could explain why the N-BAR domain of endophilin, but not its SH3 domain, is sufficient to rescue locomotion defects in endophilin-depleted mutants in Caenorhabidis elegans [25] . Altogheter, our findings confirm that besides the well-accepted contribution of SH3-mediated interactions, PI clustering induced by N-BAR domains has a major role in the downstream recruitment of proteins, such as dynamin. Although the formation of PI micro-domains was recently reported for several BAR domains [26] , our numerical simulations importantly show that PtdIns(4,5)P 2 molecules clustered by the BIN1 N-BAR domain are not sequestered ( Fig. 8d ). Therefore, clustered PIs could still be available to interact with downstream partners containing PI-binding motifs. The fact that a similar behaviour was observed at an initial physiologically relevant concentration, that is, 1% PtdIns(4,5)P 2 ( Supplementary Fig. 12 ), supports the potential implication of PI clustering in cell-trafficking events. This mechanism appears to be a general property of proteins that interact with PIs. The ANTH domain of AP180 and the ENTH of Epsin2 are also capable to cluster PtdIns(4,5)P 2, and thus, locally concentrate PI-binding motifs on membranes ( Fig. 7 ). Our experimental observations and CG simulations show that PtdIns(4,5)P 2 clustering occurs on flat membranes, although membrane curvature substantially amplifies the effect. In agreement with our experimental observations and CG simulations, theoretical studies have shown that the interaction of a positively charged protein with an oppositely charged membrane not only involves electrostatic interactions, but also an entropic effect that may lead to lipid demixing near the protein surface [23] . As shown experimentally, this effect is almost negligible in the case of monovalent lipids, where the fast association ( K on ) and dissociation ( K off ) rates between the protein and the membrane do not allow charged lipids to segregate [27] . However, for multivalent lipids such as PtdIns(4,5)P 2 , transient interactions produce an electrostatic potential well, reducing the dissociation rate and consequently protein diffusion, thus, allowing for a transitory segregation of PtdIns(4,5)P 2 (ref. 27 ). It is thus likely that curvature will amplify this effect, as curvature significantly reduces protein diffusion [28] and also affects lipids dynamics [26] . Under such conditions, one would expect that the transient segregation of PtdIns(4,5)P 2 generates a positive feedback, allowing proteins that selectively interact with PtdIns(4,5)P 2 to locally accumulate on PtdIns(4,5)P 2 -enriched areas, independently of their ability to polymerize (that is, AP180 and Epsin2). Nevertheless, our experiments and numerical simulations show that, on a flat membrane, the local PtdIns(4,5)P 2 concentration reaches at least three times the initial amount of PtdIns(4,5)P 2 ( Figs 7c and 8c ). Therefore, the selection of downstream partners on BIN1-induced PI clustering is likely to rely on at least a threefold increase in the local accessible PtdIns(4,5)P 2 pool. In conclusion, our observations indicate distinct roles for the N-BAR and the SH3 domains of BIN1. The N-BAR domains facilitates dynamin recruitment through PtdIns(4,5)P 2 clustering, whereas the SH3 domain ensures dynamin accumulation and further polymerization on membranes. This observation may explain the fact that all BIN1-mutated variants in the autosomal form of CNMs (D151N and SH3-ΔC) display a similar phenotype in dynamin binding [4] . Our work also shows that clustering of PIs could be a general property of proteins containing N-BAR or PI-interacting motifs (ANTH/ENTH), as previously suggested by biophysical experiments on model membranes [27] . In addition to local PI synthesis by specific kinases and phosphatases [29] , this mechanism could be important for the spatiotemporal selection of downstream partners of PI-binding proteins, for instance, during clathrin-mediated endocytosis [3] , [30] . Lipids Natural and synthetic phospholipids, including POPS (1-palmitoyl-2-oleoyl-sn-glycero-3-phospho-L-serine), and PE (phosphatidylethanolamine)-carboxy-fluorescein are from Avanti Polar Lipids, Inc. Fluorescent GloPIPs BODIPY-TMR-PtdIns(4,5)P 2 -C 16 (GloPIP 2 ), POPC (1-palmitoyl-2-oleoyl-sn-glycero-3-phosphocholine) and POPE (1-palmitoyl-2-oleoyl-sn-glycero-3-phosphoethanolamine) are from Echelon Biosciences, Inc. TRITC-DHPE is from Avanti Polar Lipids, Inc. Alexa Fluor 488 and 647 Maleimide-labelling kits are from Invitrogen. Monoclonal mouse antibody to BIN1 (clone 99D against exon 7) is from Sigma-Aldrich and rabbitpolyclonal antibody (Ab-1) to glutatione S-transferase (GST) is from Millipore. Constructs pGEX vector coding for GST-BIN1 isoform 8 (M-Amphiphysin2), GST-BIN1 isoform 8 Q573X (SH3-ΔC), N-BAR+PI and N-BAR sequences of BIN1 were obtained as in ref. 17 . cDNA for BAR D151N (amino acid 1–255) sequences from BIN1 were obtained after cloning into pENTR1A Gateway entry vector (Invitrogen) and recombined into pGEX4T3 (N-terminal GST fusion). All constructs were confirmed by sequencing. pGEX vectors coding for GST-PH OSH2 and GST-PH PLCδ were a kind gift from Mark Lemmon (University of Pennsylvania). pGEX-PHD2x ING2 was described elsewhere [12] . pEGFP-BIN1 D151N and pEGFP-BIN1 K575X (SH3-ΔC) were obtained as in ref. 4 . pEGFP BIN1 isoform 8 was obtained from P. De Camilli (Yale University, New Haven), mCherry-PH(PLCδ) and mCherry-Dynamin were kindly provided by Arnaud Echard (Institut Pasteur, Paris) and Christien Merrifield (LEBS, Gif-sur-Yvette), respectively. Transfection and microscopy HeLa cells (CCL2 from ATCC) were seeded on glass coverslips overnight. Cells were then transfected for 18 h with full-length GFP-BIN1, GFP-BIN1 D151N, GFP-BIN1 K575X, mCherry-PH(PLCδ) and mCherry-Dynamin using x-tremGENE9 (Roche). Fixed cells were obtained after incubation with 4% paraformaldehyde for 20 min at room temperature, washed with phosphate-buffered saline (PBS), incubated with PBS-0.1 M NH 4 Cl for 5 min and then washed with PBS. Fixed cells were visualized using a Leica DMRA and a CoolSnapHQ2 camera, × 100 objective numerical aperture 1.25 oil Ph 3 CS (HCX PL APO) and analyzed with the Metamorph software. Three-dimensional stacks were acquired and deconvolved to build a projection on one plane using Image J. Images are presented as a z-projection of all planes. Three-dimensional visualization of GFP-BIN1 or mCherry-PH(PLCδ) was performed by surface rendering (Imaris; Bitplane) of 13 z-planes. For live-cell imaging, glass coverslips were mounted on a Ludin imaging chamber after 18 h transfection. Imaging was performed on a Spinning disk microscope based on a CSU-X1 Yokogawa head mounted on an inverted Ti-E Nikon microscope equipped with a motorized XY Stage. Images were acquired through a × 100 objective numerical aperture 1.4 Plan-Apo objective with a Photometrics Coolsnap HQ2 CCD camera. Optical sectioning was performed using a piezo stage (Mad City Lab). A dual Roper/Errol laser lounge equipped with 491 and 561 nm laser diodes (50 mW each) and coupled to the spinning disk head through a single fibre was used. Multi-dimensional acquisitions were performed in streaming mode using Metamorph 7 software. Images were collected every second (500 msec exposure). Protein purification and fluorescent labelling Human recombinant isoforms of amphiphysin (1, 2 and BIN1 mutant Q573X) and N-BAR domains were expressed in Rosetta 2 bacteria and purified by affinity chromatography using glutathione Sepharose 4B beads according to the manufacturer’s instructions (GE Healthcare) in 50 mM Tris at pH 8.0, 100 mM NaCl. Proteins were expressed overnight at 18 °C using 1 mM IPTG. Proteins were then dialyzed overnight in a Slide-A-Lyzer dialysis cassette (MWCO 10,000) before Alexa Fluor 488 or 647 maleimide labelling, following the protocol described by the manufacturer (Invitrogen). Protein concentrations were measured using a Bradford assay (Biorad). Recombinant GST-tagged proteins corresponding to the different PI-binding motifs (PH-domain of PLCδ, PH-domain of OSH2 and PHD domain of ING2) were expressed in Escherichia coli strain BL21(DE3) and purified by affinity chromatography as above described. All proteins were expressed for 3 h at 37 °C using 0.2 mM IPTG except for the tandem PHD domain of ING2, which was produced overnight at 22 °C with 0.1 mM IPTG. PI-binding domains were labelled by conjugation of amine-reactive Alexa Fluor 647 carboxylic acid succinimidyl ester (Invitrogen). In brief, proteins were dialyzed against 0.1 M sodium bicarbonate buffer (pH 6.9) containing 100 mM NaCl and concentrated to 2 mg ml −1 . Proteins were then incubated with 5 M excess of AlexaFluor 647 carboxylic acid succinimidyl ester (dissolved in DMSO) for 1 h at room temperature on a rotating wheel. Each conjugate was chromatographed on a PD-10 desalting column (Amersham Biosciences) in PBS at pH 7.4. The separation of the labelled protein from the free dye was followed using a UV lamp. The labelling and purity of the proteins and the absence of free dye were checked by sodium dodecyl sulfate polyacrylamide gel electrophoresis and coomassie staining. Labelled proteins were concentrated versus a PBS solution (pH 7.4). Recombinant dynamin was produced in Sf9 cells using the Baculogold system, then purified and labelled following a previously published protocol [13] . Epsin2 was expressed in baculovirus and AP180 in BL21/DH3a cells and purified by GST pull down as described in ref. 20 . Proteins were cleaved by PreScission protease and then labelled with Alexa Fluor 488 C5 maleimide (Invitrogen). All proteins were stored in Hepes 20 mM at pH=7.4, NaCl 100 mM, MgCl 2 1 mM. Finally, glycerol was added to 10% final and all proteins were flash frozen in liquid N 2 . Flat membrane experiments Flat membrane sheets experiments were adapted from Itoh et al . [7] In contrast with other model systems (see for instance [31] ) flat membrane sheets a priori allows to precisely tune the amount of PIs incorporated in the membrane, as the final membrane lipid composition should not differ from that of the initial lipid mixture. Lipid solutions were prepared to a final concentration of 10 mg ml −1 in chloroform. Lipid mixtures consisted of a plasma membrane-like mixture composition following [32] with a molar proportion of: 40% egg phosphatidylcholine, 20% liver phosphatidylethanolamine, 25% brain sphingomyelin, 15% brain phosphatidylserine and a molar ratio of 1:1 of cholesterol. The amount of total negatively charged lipids was kept to 15% for any of the mixtures containing PIs (brain phosphatidylinositol-4,5-bisphosphate, brain phosphatidylinositol-4 monophosphate or 1,2-dioleoyl- sn -glycero-3-phospho-(1′-myo-inositol-5′-phosphate)) at the expenses of brain phosphatidylserine. Fluorescent GloPIP 2 was added to 0.01%. To prepare flat membranes, we deposited two 1-μl droplets of the corresponding lipid solution on a 22 × 44 mm clean glass coverslip. Coverslips were kept under vacuum overnight to ensure total evaporation of any trace of chloroform. Lipids were pre-hydrated for 30 min in an incubator (37 °C, 10% CO 2 and 100% humidity). Coverslips were then mounted as in ref. 7 and hydrated by injecting 15 μl of buffer (10 mM Tris, pH 7.4, 100 mM NaCl and 0.1 mg ml −1 of casein). Flat membranes were imaged on a confocal A1R Ti-Eclipse inverted microscope. Liposome flotation assays Liposomes of various lipid compositions (60% POPC, 28% POPE, 2% PE-carboxyfluorescein and 10% POPS (control) or 5% POPS and 5% PIs) were prepared by mixing chloroform stocks and incubated 10 min at 37 °C to homogenize lipids. Lipids were then evaporated for 1 h under nitrogen to form a dried film and placed in a vacuum chamber for 2 h to eliminate traces of solvent. The lipid mixtures were resuspended in PBS (Sigma-Aldrich) preheated at 37 °C to give 1 mM lipid suspensions and hydrated for 1 h in a 37 °C water bath with vigourous vortexing every 10 min. Lipid suspensions were submitted to five cycles of freezing and thawing using liquid nitrogen and a water bath (37 °C). Lipid suspensions were then sonicated for 30–60 min in a water bath and extruded 21 times using an Avanti Mini-extruder with 30 nm polycarbonate filters (to give 30–38 nm liposomes) or extruded with 100 nm polycarbonate filters (to give ~120 nm liposomes). The size distribution of the liposomes was determined by dynamic light scattering (Dynapro). Protein and liposomes ((1 μg protein (between 0.18 and 0.25 μM) and 200 μM total lipids (5 μM PIP accessible) for PI-binding specificity)) were incubated 20 min in 100 μl PBS at room temperature in polycarbonate tubes (adapted to a TLA 100.2 Beckman rotor). The protein–lipid suspensions were adjusted to 30% w vol −1 sucrose (in PBS) by adding and mixing 100 μl of 60% sucrose in PBS and overlaid with two cushions: 250 μl of 25% sucrose (in PBS) and 50 μl of PBS with no sucrose. The tubes were then centrifuged at 200,000 g for 1 h at 20 °C (TL 100, Beckman) (during centrifugation, the fluorescent liposomes migrate to the top buffer layer). After ultracentrifugation, fractions were collected from bottom to top using aHamilton syringe and the last top fluorescent fractions were analyzed with immunoblotting using an anti-GST antibody. Quantifications were done using the Image Lab software (Bio-Rad). Image processing and quantification Line profiles of the fluorescence intensities were done using Image J and the kymographs were made using the Kymograph plugin ( http://www.embl.de/eamnet/html/body_kymograph.html ). Protein binding was quantified by measuring the mean grey value of a 200 × 200 pixels square. This square was placed on a representative image region, covering both the membrane bulk (that is, the lamellae) and BIN1, AP180 and Epsin-positive structures. The mean gray values of the protein intensity was normalized by the mean gray value of the membrane intensity (as indicated by Glo-PIP 2 fluorescence) in the same selected region, to correct for the heterogeneous distribution of membrane stacks through the sample. Mean gray values were measured once the steady-state of protein binding was reached, which was estimated from the binding kinetics to be ≥900 s. Protein binding was averaged from at least three independent experiments. Mean gray values were mesured using Image J. The amount of fluorophore and confocal parameters were kept constant between experiments and samples. The fluorescence backrgound corresponding to the membrane and the protein intesnsity, respectively, was substracted by performing a cross-section analysis of several representative regions in each image displaying non-binding events using Image J. As illustrated in Supplementary Fig. 2d and detailed below, the total fluorescence intensities measured from both channels ( I cyan and I red ) in region R 4 correctly reports protein accumulation. In region R 4 , protein binding is measured as R 4 = I cyan / I red =( I lamellae cyan + I tube cyan )/( I lamellae red + I tube red ), where I lamellae cyan and I tube cyan are the background-subtracted fluorescence signals from the protein channel (cyan) in the lamellae and in the tubule zones of region R 4, respectively and I lamellae red and I tube red are the same values from the membrane channel (red). Because the amount of lipids available for protein binding is much smaller in the tubulated zone of region R 4 than in the lamella zone of region R 4 , I tube red is much smaller than I lamellae red and R 4 ~ I lamellae cyan / I lamellae red + I tube cyan / I lamellae red . The first term corresponds to the protein binding in the lamella zone of region R 4 . Because BIN1 binding does not induce any significant change in the binding of the PIP 2 -probe in the lamella region ( R 1 = I lamellae cyan / I lamellae red ~ R 2 , Supplementary Fig. 2d ), the second term represents the increase in PIP 2 -probe binding due to the presence of BIN1-induced tubules and normalized by the same factor as in the lamellae ( I lamellae red ). Dynamin recruitment curves were fitted using Origin software according to the Hill equation. Fitting was performed by imposing a cooperative Hill coefficient of n H =3, which corresponds to the value obtained for the best fit of dynamin under control conditions. Curves correspond to at least three independent experiments. Statistical analyses Results are shown as a box plot where the means (solid square)±s.e. (s.d.) and median (solid line) are displayed, except indicated otherwise. Average values displayed correspond to at least three independent experiments. Statistical significance was assessed using student’s t -test with P values are denoted by * P <0.01, ** P <0.01, *** P <0.001. MD simulations All MD simulations were performed using the software GROMACS 4 (ref. 33 ) and are based on the MARTINI force field [34] . The force field for PtdIns(4,5)P 2 lipids was developed following the basic MARTINI strategy, starting from the available force field for PdtIns(3,4)P 2 by (i) replacing one of the two palmitoyl acyl chains with an arachidonoyl acyl chain, (ii) connecting each of the three phosphate beads with one of the three distinct beads forming the inositol ring and (iii) describing the three beads forming the inositol ring with polar ‘P1’ particles. Non-bonded interactions (electrostatics and Lennard–Jones) were treated using shifted potentials with a cutoff radius of 1.2 nm. Pressure and temperature were controlled through the coupling to an external bath using the velocity rescale thermostat [35] and a semi-isotropic Berendsen barostat [36] ; temperature was kept at 300 K in all systems. A time step of 10 fs was used and a standard time conversion factor of 4 [34] was used to estimate the length of all production and equilibration runs. The lipid bilayer used in the simulations was generated via spontaneous self-assembly of a small lipid patch that was subsequently replicated to reach the desired size of ~22 × 22 nm. The final bilayer consisted of 1,440 lipids, symmetrically distributed between the two leaflets, with the following concentrations: 80% POPC, 15% POPS, 5% PtdIns(4,5)P 2 . The three protein domains used in the study are the homodimeric N-BAR domain of amphiphysin (PDB: 1URU) [1] , the monomeric ANTH domain of AP180 (PDB: 1HFA) [21] and the monomeric ENTH domain of Epsin2 (PDB: 1H0A) [37] . The CG parameters (coordinates, topology) for the three proteins were obtained using an automated procedure, whereas protein secondary structure was restrained to the crystallographic conformation [38] . In all simulations, a single protein was initially positioned between 6 and 10 nm away from the lipid bilayer, and the system was solvated with CG water beads. Counter-ions were then added to neutralize the system. The overall system size was ~22 × 22 × 20 nm 3 . After solvation, the systems were subject to 500 steps of energy minimization and, whenever necessary, to a short MD run (5 ns) performed with a time step of 2 fs. Next, an ensemble of five simulations for each system (N-BAR, ANTH and ENTH) was started from the same coordinates but different initial velocities. All simulations were run for 4 μs. Analyses presented in the text were carried out over the last 2 μs of each simulation. Similar simulations were performed after replacement of the protein with four unfolded polylysine motifs (sequence: KKKKKKKK), initially positioned ~6 nm away from the lipid bilayer. Three independent simulations of 4 μs were carried out. Two additional simulations of 20 μs each were carried out in the presence of a N-BAR homodimer, after doubling the membrane size along the x-direction. The two simulations were carried out, respectively, at a 5 and 1% PtdIns(4,5)P 2 concentration. The second system was obtained from the first by manually changing the excess PtdIns(4,5)P 2 lipids in POPS lipids and by adjusting the number of counter-ions. In these simulations, the phase-space accessible to the protein was limited along the x direction by imposing a lower and an upper wall to the motion of its center of mass. In practical terms, this was achieved by an external restraining potential, as implemented in the software suite PLUMED [39] , and that is different from zero only when the x-coordinate of the protein center of mass falls outside a specific range. In our case, the protein domain was allowed to sample only half of the available phase space along the x-coordinate, and the resulting PtdIns(4,5)P 2 concentration in the half of the simulation box in which the protein was confined was then plotted as a function of time ( Fig. 8e and Supplementary Fig. 12 ). Lipid clustering was assessed by either computing the radial distribution function of the various lipids using the center of mass of the protein as a reference ( Supplementary Fig. 9 ) or by computing the two-dimensional number density of lipids within the membrane plane after fitting the trajectory using the protein as a reference ( Fig. 8a ). The local increase in PtdIns(4,5)P 2 percentage as a function of N-BAR bound density ( Fig. 8c ) was computed by assuming that each N-BAR homodimer is bound to 18±1 PtdIns(4,5)P 2 lipids ( Fig. 8b ) and by estimating its surface area as 60 nm 2 . The resulting local percentage as a function of protein bound density is then estimated by simply weighted averaging the percentage of PtdIns(4,5)P 2 lipids in the free membrane surface (5% concentration) and in the N-BAR bound membrane surface (18% concentration), considering that the area per lipid computed in the simulations is of ~0.60 nm 2 . All molecular images were rendered with Visual Molecular Dynamics (VMD) [40] . How to cite this article: Picas, L. et al. BIN1/M-Amphiphysin2 induces clustering of phosphoinositides to recruit its downstream partner dynamin. Nat. Commun. 5:5647 doi: 10.1038/ncomms6647 (2014).